VE-PTP regulates VEGFR2 activity in stalk cells to establish endothelial cell polarity and lumen formation Vascular endothelial growth factor (VEGF) guides the path of new vessel sprouts by inducing VEGF receptor-2 activity in the sprout tip. In the stalk cells of the sprout, VEGF receptor-2 activity is downregulated. Here, we show that VEGF receptor-2 in stalk cells is dephosphorylated by the endothelium-specific vascular endothelial-phosphotyrosine phosphatase (VE-PTP). VE-PTP acts on VEGF receptor-2 located in endothelial junctions indirectly, via the Angiopoietin-1 receptor Tie2. VE-PTP inactivation in mouse embryoid bodies leads to excess VEGF receptor-2 activity in stalk cells, increased tyrosine phosphorylation of VE-cadherin and loss of cell polarity and lumen formation. Vessels in ve-ptp −/− teratomas also show increased VEGF receptor-2 activity and loss of endothelial polarization. Moreover, the zebrafish VE-PTP orthologue ptp-rb is essential for polarization and lumen formation in intersomitic vessels. We conclude that the role of Tie2 in maintenance of vascular quiescence involves VE-PTP-dependent dephosphorylation of VEGF receptor-2, and that VEGF receptor-2 activity regulates VE-cadherin tyrosine phosphorylation, endothelial cell polarity and lumen formation. Vascular endothelial growth factor (VEGF)-A (henceforth, denoted as VEGF) is essential for blood vessel development during embryogenesis, for angiogenesis in the adult and for regulation of vascular permeability [1] . VEGF binds to two receptor tyrosine kinases, VEGFR1 and VEGFR2. Whereas VEGFR1 primarily serves a negative regulatory role, VEGFR2 transduces all known effects of VEGF [2] . Gene targeting of vegfa and vegfr2 both result in early embryonic lethality due to arrested endothelial cell (EC) differentiation [3] , [4] , [5] . Binding of VEGF to VEGFR2 induces receptor dimerization, activation of the kinase and autophosphorylation of tyrosine residues [6] , [7] . Autophosphorylated residues regulate kinase activity and bind signal transducers that propagate signals eventually resulting in EC survival, proliferation, migration and lumen formation. Kinase activity is tightly regulated, for example, through protein tyrosine phosphatases (PTPs). Vascular endothelial (VE) protein tyrosine phosphatase (VE-PTP in the mouse; PTP-receptor beta; PTP-RB in the human) is specifically expressed in ECs [8] , [9] . Inactivation of the ve-ptp gene results in normal vasculogenesis, but abnormal angiogenesis and failure to organize the vasculature into higher-order branched vessels, leading to embryonic death at E11 (ref. 8 , 9 ). VE-PTP dephosphorylates substrates at EC junctions, such as the receptor tyrosine kinase Tie2 (ref. 10 ), and adherens junction components VE-cadherin [11] and its partner plakoglobin [12] . Tie2, and its activating ligand Angiopoietin-1 (Ang1) are required for vessel integrity [13] . Ang1 promotes formation of Tie2/VE-PTP complexes at cell–cell contacts, thereby regulating junctional stability [14] . Phosphorylation of VE-cadherin is accompanied by loosening of adherens junctions and vascular permeability. VE-cadherin silencing or gene targeting in vitro [15] , in zebrafish [16] and in mice [17] disturb endothelial polarization and vessel lumen formation. Interactions between VE-cadherin and PAR3 and PAR6, members of the cell polarity complex [18] , [19] , may be critical for the polarization and lumen formation processes. We have previously shown that VE-PTP associates with and dephosphorylates VEGFR2 (ref. 20 ). We now show that VE-PTP regulates junctional activity of VEGFR2 in a Tie2-dependent manner, accompanied by decreased VE-cadherin phosphorylation. Overall, VE-PTP serves as a molecular relay to orchestrate junctional maturation, EC polarization and lumen formation during VEGF-driven sprouting angiogenesis. Angiogenic sprouting in VE-PTP-deficient embryoid bodies We analysed sprouting angiogenesis in mouse embryoid bodies (EBs) from wild-type (WT) and ve-ptp −/− embryonic stem cells (ESCs) [8] , [21] . Ve-ptp −/− EBs formed a denser network of vessel sprouts with similar length but with increased area compared with WT EBs ( Fig. 1a–c ). There was a tenfold increase in CD31/VE-cadherin double-positive ECs in VEGF-treated ve-ptp −/− EBs compared with VEGF-treated wild-type EBs ( Fig. 1d ). Moreover, the ve-ptp −/− ECs extended numerous long filopodia throughout the sprout, while most WT stalk cells did not ( Fig. 1e ). We hypothesized that increased EC proliferation and filopodia formation might be due to elevated VEGFR2 activity. 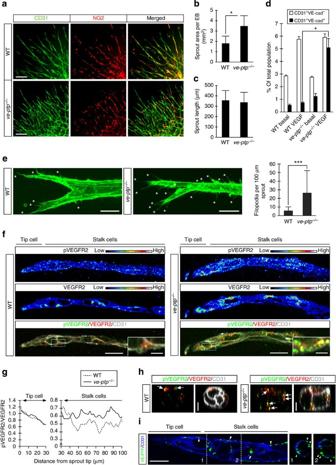Figure 1: VEGFR2 stalk cell activity inve-ptp−/−EBs. WT andve-ptp−/−EBs cultured in 3D collagen gels with VEGF (20 ng ml−1) until day 14, unless otherwise indicated. (a) Immunostaining of ECs (CD31; green) and pericytes (NG2; red) in WT andve-ptp−/−EBs. Scale bars; 100μm. (b) Quantification of CD31-positive sprout area per EB. Mean±s.d.,n=6 EBs per genotype. *P<0.05,t-test. (c) Quantification of sprout length, from core to sprout tip. Mean±s.d.,n=100 sprouts per genotype. (d) Flow sorting of dissociated WT andve-ptp−/−EBs (day 9; 2D culture) identified CD31 and VE-cadherin double-positive ECs. Mean±s.d.,n=150 EBs per genotype. *P<0.05,t-test. (e) Detection of CD31-positive long (> 3 μm) filopodia (asterisk) per 100 μm EB sprout length. Mean±s.d.,n=20 sprouts per genotype. ***P<0.001,t-test. (f) Representation of pY1175 VEGFR2 (upper) and VEGFR2 (middle) immunofluorescent staining using a 16-colour intensity scale. Merged image (bottom panel) shows pVEGFR2 (green), VEGFR2 (red) and CD31 (white). Scale bar; 20 μm. High-magnification insets show pVEGFR2; scale bar; 5 μm. (g) Ratio pVEGFR2/VEGFR2 fluorescent intensities per total CD31-area. Mean±s.d.,n= 7 sprouts per genotype. The mean pVEGFR2/VEGFR2 ratio differed significantly between WT and ve-ptp−/−stalk cell region of the sprout;P<0.001 as determined using paired two-tailedt-test. (h) Vertical-view image of WT andve-ptp−/−sprouts immunostained for pY1175 VEGFR2 (green), VEGFR2 (red) and CD31 (white). Arrows indicate pVEGFR2. Scale bars; 5 μm. (i) Immunostaining for VE-PTP (green) and CD31 (blue) in WT sprouts, show localization of VE-PTP in junctions (arrowheads) in the stalk region. Broken lines in the left, larger panel indicate position of vertical-view images shown in panels to the right. Scale bar; 20 μm. All analyses were repeated at least three times. Figure 1: VEGFR2 stalk cell activity in ve-ptp −/− EBs. WT and ve-ptp −/− EBs cultured in 3D collagen gels with VEGF (20 ng ml −1 ) until day 14, unless otherwise indicated. ( a ) Immunostaining of ECs (CD31; green) and pericytes (NG2; red) in WT and ve-ptp −/− EBs. Scale bars; 100μm. ( b ) Quantification of CD31-positive sprout area per EB. Mean±s.d., n =6 EBs per genotype. * P <0.05, t -test. ( c ) Quantification of sprout length, from core to sprout tip. Mean±s.d., n =100 sprouts per genotype. ( d ) Flow sorting of dissociated WT and ve-ptp −/− EBs (day 9; 2D culture) identified CD31 and VE-cadherin double-positive ECs. Mean±s.d., n =150 EBs per genotype. * P <0.05, t -test. ( e ) Detection of CD31-positive long (> 3 μm) filopodia (asterisk) per 100 μm EB sprout length. Mean±s.d., n =20 sprouts per genotype. *** P <0.001, t -test. ( f ) Representation of pY1175 VEGFR2 (upper) and VEGFR2 (middle) immunofluorescent staining using a 16-colour intensity scale. Merged image (bottom panel) shows pVEGFR2 (green), VEGFR2 (red) and CD31 (white). Scale bar; 20 μm. High-magnification insets show pVEGFR2; scale bar; 5 μm. ( g ) Ratio pVEGFR2/VEGFR2 fluorescent intensities per total CD31-area. Mean±s.d., n = 7 sprouts per genotype. The mean pVEGFR2/VEGFR2 ratio differed significantly between WT and ve-ptp −/− stalk cell region of the sprout; P <0.001 as determined using paired two-tailed t -test. ( h ) Vertical-view image of WT and ve-ptp −/− sprouts immunostained for pY1175 VEGFR2 (green), VEGFR2 (red) and CD31 (white). Arrows indicate pVEGFR2. Scale bars; 5 μm. ( i ) Immunostaining for VE-PTP (green) and CD31 (blue) in WT sprouts, show localization of VE-PTP in junctions (arrowheads) in the stalk region. Broken lines in the left, larger panel indicate position of vertical-view images shown in panels to the right. Scale bar; 20 μm. All analyses were repeated at least three times. Full size image Indeed, immunostaining for VEGFR2 and the VEGFR2 phosphorylation site pY1175 ( Fig. 1f ) showed increased levels in ve-ptp −/− sprouts compared with WT ( Fig. 1g ). The pVEGFR2/total VEGFR2 ratio was significantly higher in the ve-ptp −/− stalks compared with WT stalks. The pVEGFR2 activity often colocalized with CD31 immunostaining, which was used to identify EC junctions ( Fig. 1h ). The VEGFR2 and pVEGFR2 stainings did not always colocalize, possibly because the antibodies against pVEGFR2 and VEGFR2 detected receptor intra- and extracellular domains, respectively. Immunostaining for VE-PTP also showed junctional localization ( Fig. 1i ). Supplementary Figure S1a,b shows that VE-PTP ablation was accompanied by reduced pericyte coating, indicating immature sprouts. Moreover, whereas ve-ptp transcripts were efficiently eliminated after gene targeting, there was no change in expression levels of genes known to affect angiogenic sprouting, such as delta-like 4 , notch 1 and vegfr2 ( Supplementary Fig. S1c–f ). VE-PTP dephosphorylates VEGFR2 in a Tie2-dependent manner Substrates for VE-PTP include Tie2, an angiopoietin receptor implicated in control of vascular quiescence [13] . Lack of Ang1 or Tie2 leads to disturbed vascular remodelling during mouse embryonic development [22] , [23] , [24] . To compare VE-PTP’s effect on VEGFR2 and Tie2, we employed a substrate-trapping, phosphatase-dead mutant of VE-PTP (D/A VE-PTP; aspartic acid 1180 in the catalytic domain exchanged for alanine). Substrate-trapping mutants bind their substrates without dephosphorylation [25] . Accordingly, expression of D/A VE-PTP allowed co-immunoprecipitation of pY992Tie2 with VE-PTP in Ang1-treated cells ( Fig. 2a ). Tie2 was co-immunoprecipiated also with WT VE-PTP, which was enzymatically active towards a standard substrate, Src optimal peptide ( Supplementary Fig. S2a ). The pY992Tie2 signal in response to Ang1 was weaker in cells expressing WT VE-PTP than D/A VE-PTP, indicating dephosphorylation of phosphorylated Tie2 by WT VE-PTP ( Fig. 2a ). Tie2 was also dephosphorylated in vitro using a purified VE-PTP catalytic domain fragment ( Supplementary Fig. S2b ). 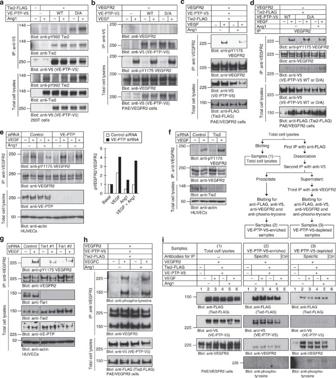Figure 2: VE-PTP dephosphorylates VEGFR2 in a Tie2-dependent manner. HEK 293 T cells, PAE/VEGFR2 or HUVECs treated as indicated with VEGF (20 ng ml−1, 15 min) or Ang1 (200 ng ml−1, 30 min) or VEGF+Ang1 (Ang 1, 200 ng ml−1, 15 min, followed by addition of VEGF 20 ng ml−1, 15 min). Analyses were performed by immunoblotting (blot) on total cell lysates or on immunoprecipitations (IPs) as indicated. All experiments were repeated at least twice. (a) HEK 293T cells expressing FLAG-tagged Tie2 (Tie2-FLAG) and WT or D/A mutant V5-tagged VE-PTP (VE-PTP-V5), treated with Ang1. (b) PAE/VEGFR2 cells expressing WT or D/A mutant VE-PTP-V5, treated with VEGF. (c) PAE/VEGFR2 cells expressing VE-PTP-V5 and Tie2-FLAG, treated with VEGF and Ang1. (d) PAE/VEGFR2 cells expressing WT VE-PTP-V5, D/A VE-PTP-V5 and Tie2-FLAG, treated with VEGF and Ang1. (e) HUVECs transfected with control or VE-PTP siRNAs, treated with VEGF and Ang1. Quantification of pVEGFR/VEGFR2 levels (right). (f) HUVECs transfected with control or Tie2 siRNAs, treated with VEGF. (g) HUVECs transfected with control siRNA or with two different Tie1 siRNAs (#1 and #2), and treated with VEGF. Samples were run on the same gel/blot. (h) PAE/VEGFR3 cells expressing VE-PTP-V5 and Tie2-FLAG, treated with 200 ng ml−1VEGFC, for 15 min. (i) PAE/VEGFR2 cells expressing VE-PTP-V5 and Tie2-FLAG (Tie2-F), treated with VEGF and Ang1 individually and in combination. Sequential IP was performed first with anti-FLAG antibodies followed by low pH elution and re-IP with anti-V5 antibodies (resulting in VE-PTP enriched samples) as outlined to the upper right. The supernatants (VE-PTP-depleted samples) were used for re-IP with anti-VEGFR2 antibodies. Immunoblotting was performed of total cell lysates (Sample 1; left panel), VE-PTP-V5-enriched samples (Sample 2; middle panel) and VE-PTP-depleted samples (Sample 3; right panel). For the VE-PTP enriched and depleted samples, lanes 1–5 show the results of IP with specific antibodies; control IgG was used for IP of sample 6. Figure 2: VE-PTP dephosphorylates VEGFR2 in a Tie2-dependent manner. HEK 293 T cells, PAE/VEGFR2 or HUVECs treated as indicated with VEGF (20 ng ml −1 , 15 min) or Ang1 (200 ng ml −1 , 30 min) or VEGF+Ang1 (Ang 1, 200 ng ml −1 , 15 min, followed by addition of VEGF 20 ng ml −1 , 15 min). Analyses were performed by immunoblotting (blot) on total cell lysates or on immunoprecipitations (IPs) as indicated. All experiments were repeated at least twice. ( a ) HEK 293T cells expressing FLAG-tagged Tie2 (Tie2-FLAG) and WT or D/A mutant V5-tagged VE-PTP (VE-PTP-V5), treated with Ang1. ( b ) PAE/VEGFR2 cells expressing WT or D/A mutant VE-PTP-V5, treated with VEGF. ( c ) PAE/VEGFR2 cells expressing VE-PTP-V5 and Tie2-FLAG, treated with VEGF and Ang1. ( d ) PAE/VEGFR2 cells expressing WT VE-PTP-V5, D/A VE-PTP-V5 and Tie2-FLAG, treated with VEGF and Ang1. ( e ) HUVECs transfected with control or VE-PTP siRNAs, treated with VEGF and Ang1. Quantification of pVEGFR/VEGFR2 levels (right). ( f ) HUVECs transfected with control or Tie2 siRNAs, treated with VEGF. ( g ) HUVECs transfected with control siRNA or with two different Tie1 siRNAs (#1 and #2), and treated with VEGF. Samples were run on the same gel/blot. ( h ) PAE/VEGFR3 cells expressing VE-PTP-V5 and Tie2-FLAG, treated with 200 ng ml −1 VEGFC, for 15 min. ( i ) PAE/VEGFR2 cells expressing VE-PTP-V5 and Tie2-FLAG (Tie2-F), treated with VEGF and Ang1 individually and in combination. Sequential IP was performed first with anti-FLAG antibodies followed by low pH elution and re-IP with anti-V5 antibodies (resulting in VE-PTP enriched samples) as outlined to the upper right. The supernatants (VE-PTP-depleted samples) were used for re-IP with anti-VEGFR2 antibodies. Immunoblotting was performed of total cell lysates (Sample 1; left panel), VE-PTP-V5-enriched samples (Sample 2; middle panel) and VE-PTP-depleted samples (Sample 3; right panel). For the VE-PTP enriched and depleted samples, lanes 1–5 show the results of IP with specific antibodies; control IgG was used for IP of sample 6. Full size image In contrast, expression of WT and D/A VE-PTP in VEGFR2-expressing Porcine aortic endothelial (PAE) cells lacking Tie2 expression did not allow co-immunoprecipitation of VEGFR2 with VE-PTP ( Fig. 2b ). The level of VEGFR2 phosphorylation remained unaffected by VE-PTP, in accordance with previous data [20] , [26] . However, immunoprecipitated pVEGFR2 was efficiently dephosphorylated in vitro , by the purified VE-PTP catalytic fragment ( Supplementary Fig. S2b ). Importantly, introduction of Tie2 together with VE-PTP and VEGFR2 in the PAE cells, followed by treatment with VEGF+Ang1, allowed VE-PTP-mediated pVEGFR2 dephosphorylation ( Fig. 2c ; Supplementary Fig. S3a,b ). VEGFR2 moreover formed a complex with the D/A VE-PTP mutant in the presence of Tie2, in particular, in response to the combination of ligands ( Fig. 2d ). The protection by D/A VE-PTP of VEGFR2 from dephosphorylation was poor, possibly indicating that VEGFR2 was co-precipitated indirectly, via a D/A VE-PTP/Tie2 complex and therefore exposed to the action of other cellular phosphatases. The requirement for Tie2 in VE-PTP dependent dephosphorylation of VEGFR2 was further demonstrated by silencing either VE-PTP or Tie2 in primary ECs using short interfering RNA (siRNA). Thus, i) silencing of VE-PTP rendered cells insensitive to Ang1’s effect on pVEGFR2 dephosphorylation ( Fig. 2e ) and ii) silencing of Tie2 increased VEGF-induced pVEGFR2 levels compared with the control ( Fig. 2f ). Combined, these results indicate that VE-PTP dephosphorylates VEGFR2 in a Tie2-dependent manner. Unlike the effect of silencing Tie2, introduction of Tie1 siRNA did not increase VEGF-induced accumulation of pVEGFR2, instead, there was a further decrease in pVEGFR2 levels in the Tie1-silenced cells ( Fig. 2g ). These data are in accordance with a negatively regulatory role for Tie1 visavi Tie2 (ref. 27 ). Furthermore, VEGFC-induced VEGFR3 tyrosine phosphorylation was not influenced by co-expression of Tie2 ( Fig. 2h ). A Tie2-truncated mutant, retaining the transmembrane domain but lacking the intracellular part including the kinase domain, partially decreased VEGFR2 phosphorylation in an Ang1-insensitive manner ( Supplementary Fig. S3a ). Introduction of a kinase-dead (KD) Tie2 mutant [22] suppressed VEGFR2 phosphorylation to an extent similar to that seen for Ang1-treated cells expressing WT Tie2. The additional slight effect of Ang1 on cells expressing KD Tie2 seen here may reflect Tie2-independent effects of Ang1 (ref. 28 ). We conclude that Tie2 kinase activity is not required for full VE-PTP activity towards VEGFR2. We hypothesized that VE-PTP’s effect towards Tie2 and VEGFR2 may be through formation of trimeric, constitutive complexes. To investigate a potential trimeric complex, we introduced V5-tagged VE-PTP and FLAG-tagged Tie2 into PAE/VEGFR2 cells that were treated or not with VEGF and Ang1, and performed consecutive immunoprecipitation and immunoblotting. The expression levels of VEGFR2, Tie2 and VE-PTP were comparable in the different conditions ( Fig. 2i , left panel). Immunoprecipitation of Tie2 from cells expressing all three molecules followed by re-immunoprecipitation of VE-PTP allowed visualization of Tie2, VE-PTP and VEGFR2 in subsequent immunoblotting ( Fig. 2i middle panel), showing the existence of a trimeric complex. We noted that the intracellular, lower molecular weight form of VEGFR2 was included in the complex. Immunoprecipitation of VEGFR2 from the supernatant of the anti-VE-PTP re-immunoprecipitation (that is, VE-PTP-depleted), showed co-immunoprecipitation of Tie2 with VEGFR2. We conclude that VEGFR2 existed both in a constitutive complex with Tie2 alone as well as in a trimeric complex with Tie2 and VE-PTP. Furthermore, the degree of complex formation was unaffected by VEGF and Ang1. Reduced VEGFR2 phosphorylation requires cell–cell junctions VEGFR2 has been shown to colocalize and engage in complex with VE-cadherin [29] , [30] , [31] . Moreover, Tie2 accumulates at established cell–cell contacts in response to Ang1 (ref. 14 ). We asked whether VEGFR2 and Tie2 colocalized at cell–cell junctions. As seen in Fig. 3a , VEGFR2 and Tie2 translocated to cell–cell junctions in response to their respective ligand, as well as the combination of ligands (quantified in Fig. 3b ). 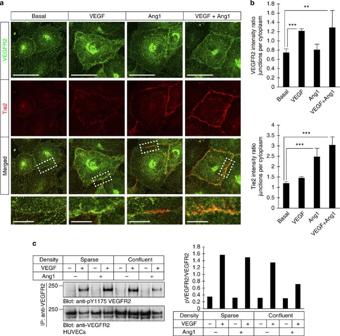Figure 3: Level of VEGFR2 phosphorylation is dependent on junctions. (a) HUVECs were pretreated with 200 ng ml−1of Ang1 (30 min), followed by addition of VEGF (20 ng ml−1, 5 min), alternatively the two ligands were used individually (Ang1 for 30 min and VEGF for 5 min). Cells were immunostained with antibodies against VEGFR2 and Tie2. Scale bars, 20 μm. High-magnification insets show VEGFR2 and Tie2 in merged images; scale bars, 5 μm. (b) Quantification of the junctional/cytoplasmic ratio of VEGFR2 (upper) or Tie2 (lower) intensities ina; mean±s.d.,n= 40–50 cells for each condition. **P<0.01. ***P<0.001,t-test. (c) Sparse and confluent HUVECs were treated with 200 ng ml−1of Ang1 (30 min), 20 ng ml−1of VEGF (15 min), individually or in combination, followed by immunoprecipitation (IP) with anti-VEGFR2 and blotting for pVEGFR2 and VEGFR2. Quantification of pVEGFR2/VEGFR2 is representative of three independent experiments. Figure 3: Level of VEGFR2 phosphorylation is dependent on junctions. ( a ) HUVECs were pretreated with 200 ng ml −1 of Ang1 (30 min), followed by addition of VEGF (20 ng ml −1 , 5 min), alternatively the two ligands were used individually (Ang1 for 30 min and VEGF for 5 min). Cells were immunostained with antibodies against VEGFR2 and Tie2. Scale bars, 20 μm. High-magnification insets show VEGFR2 and Tie2 in merged images; scale bars, 5 μm. ( b ) Quantification of the junctional/cytoplasmic ratio of VEGFR2 (upper) or Tie2 (lower) intensities in a ; mean±s.d., n = 40–50 cells for each condition. ** P <0.01. *** P <0.001, t -test. ( c ) Sparse and confluent HUVECs were treated with 200 ng ml −1 of Ang1 (30 min), 20 ng ml −1 of VEGF (15 min), individually or in combination, followed by immunoprecipitation (IP) with anti-VEGFR2 and blotting for pVEGFR2 and VEGFR2. Quantification of pVEGFR2/VEGFR2 is representative of three independent experiments. Full size image We next tested whether Ang1-dependent suppression of VEGFR2 phosphorylation required established cell–cell contacts. Indeed, VEGFR2 phosphorylation in VEGF+Ang1-treated, confluent ECs was reduced compared with treatment with VEGF alone. In sparse ECs, VEGF and VEGF+Ang1 induced similar levels of pVEGFR2 ( Fig. 3c ). In agreement, immunostaining for pVEGFR2 and VEGFR2 in confluent, VEGF-treated primary ECs showed pVEGFR2 localized to junctions after 5 and 60 min ( Supplementary Fig. S4 ). In the presence of VEGF+Ang1, junctional pVEGFR2 levels were suppressed. These results strongly suggest that VE-PTP dephosphorylates VEGFR2 via Tie2 at cell–cell junctions. To further identify the subcellular localization of VE-PTP-regulated VEGFR2, we performed in situ proximity ligation assays (PLA) using antibodies against pVEGFR2 and VEGFR2 and oligonucleotide-ligated secondary antibodies. PLA products representing phosphorylated VEGFR2 increased with VEGF and decreased with VEGF+Ang1 treatment (quantification in Fig. 4b ). Silencing of ve-ptp augmented PLA-detection of pVEGFR2 in response to VEGF; importantly, inclusion of Ang1 was without effect in VE-PTP-deficient cells. The pVEGFR2/VEGFR2 PLA spots were localized preferentially at or close to junctions in ve-ptp -silenced cells ( Fig. 4a–c ). Quantification of junctional localization showed fourfold induction of pVEGFR2/VEGFR2 in WT cells, compared with tenfold induction in ve-ptp -silenced cells. Controls for the PLA reactions ( Supplementary Fig. S5 ) by omitting primary antibodies showed a high degree of specificity. 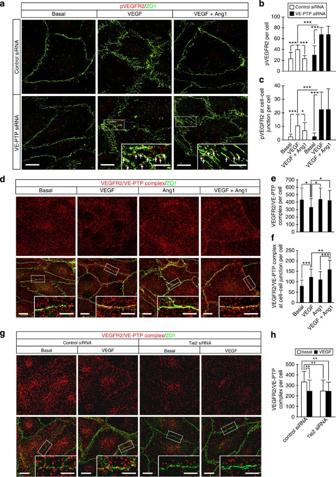Figure 4: Dephosphorylation of VEGFR2 at junctions. (a) HUVECs transfected with control orve-ptpsiRNA were stimulated with VEGF (20 ng ml−1: 60 min), and with Ang1 (200 ng ml−1; 60 min) individually or in combination, followed by PLA for pVEGFR2/VEGFR2 complexes and immunostaining with anti-ZO1 antibodies (green) to visualize cell–cell junctions. Red dots represent PLA products. Scale bars, 10 μm. High-magnification insets show PLA products at junctions; scale bars; 5 μm. (b) Quantification of number of pVEGFR2/VEGFR2 PLA products per cell. Mean±s.d.,n=45 cells per condition repeated twice. ***P<0.001,t-test. (c) Quantification of number of pVEGFR2/VEGFR2 PLA products at junctions per cell. Mean±s.d.,n= 45 cells per condition repeated twice. *P<0.05, ***P<0.001,t-test. (d) HUVECs were treated with 200 ng ml−1of Ang1 (30 min), followed by addition of 20 ng ml−1of VEGF (5 min), alternatively the two ligands were used individually (Ang1 for 30 min and VEGF for 5 min), processed and subjected to PLA using antibodies against VEGFR2 and VE-PTP and immunostaining for ZO1 (green). Scale bars, 20 μm. High-magnification insets show VEGFR2/VE-PTP PLA spots at cell–cell junctions; scale bars, 10 μm. (e) Quantification of VEGFR2/VE-PTP PLA complexes per cell. Mean±s.d.,n= 30 cells per condition. *P<0.05,t-test. (f) Quantification of VEGFR2/VE-PTP PLA complexes at junctions per cell. Mean±s.d.,n=45 cells per condition repeated twice. **P<0.01, ***P<0.001,t-test. (g) VEGFR2/VE-PTP PLA was performed in HUVECs transfected with control andtie2siRNA and treated with VEGF and Ang1 as ind, followed by PLA for VEGFR2/VE-PTP complexes, and immunostaining with anti-ZO1 antibodies. Scale bars, 20 μm. High-magnification insets show PLA products at junction; scale bars, 10 μm. (h) Quantification of VEGFR2/VE-PTP PLA complexes per cell. Mean±s.d.,n= 100 cells per condition, repeated twice. **P<0.01,t-test. Figure 4: Dephosphorylation of VEGFR2 at junctions. ( a ) HUVECs transfected with control or ve-ptp siRNA were stimulated with VEGF (20 ng ml −1 : 60 min), and with Ang1 (200 ng ml −1 ; 60 min) individually or in combination, followed by PLA for pVEGFR2/VEGFR2 complexes and immunostaining with anti-ZO1 antibodies (green) to visualize cell–cell junctions. Red dots represent PLA products. Scale bars, 10 μm. High-magnification insets show PLA products at junctions; scale bars; 5 μm. ( b ) Quantification of number of pVEGFR2/VEGFR2 PLA products per cell. Mean±s.d., n =45 cells per condition repeated twice. *** P <0.001, t -test. ( c ) Quantification of number of pVEGFR2/VEGFR2 PLA products at junctions per cell. Mean±s.d., n = 45 cells per condition repeated twice. * P <0.05, *** P <0.001, t -test. ( d ) HUVECs were treated with 200 ng ml −1 of Ang1 (30 min), followed by addition of 20 ng ml −1 of VEGF (5 min), alternatively the two ligands were used individually (Ang1 for 30 min and VEGF for 5 min), processed and subjected to PLA using antibodies against VEGFR2 and VE-PTP and immunostaining for ZO1 (green). Scale bars, 20 μm. High-magnification insets show VEGFR2/VE-PTP PLA spots at cell–cell junctions; scale bars, 10 μm. ( e ) Quantification of VEGFR2/VE-PTP PLA complexes per cell. Mean±s.d., n = 30 cells per condition. * P <0.05, t -test. ( f ) Quantification of VEGFR2/VE-PTP PLA complexes at junctions per cell. Mean±s.d., n =45 cells per condition repeated twice. ** P <0.01, *** P <0.001, t -test. ( g ) VEGFR2/VE-PTP PLA was performed in HUVECs transfected with control and tie2 siRNA and treated with VEGF and Ang1 as in d , followed by PLA for VEGFR2/VE-PTP complexes, and immunostaining with anti-ZO1 antibodies. Scale bars, 20 μm. High-magnification insets show PLA products at junction; scale bars, 10 μm. ( h ) Quantification of VEGFR2/VE-PTP PLA complexes per cell. Mean±s.d., n = 100 cells per condition, repeated twice. ** P <0.01, t -test. Full size image We also used PLA to show that VEGFR2/VE-PTP complexes were abundant in the basal condition and decreased with VEGF, as reported previously [20] ( Fig. 4d ). In response to VEGF+Ang1, the number of VEGFR2/VE-PTP complexes remained intact at the basal level when analysing the number of complexes per cell ( Fig. 4e ). However, the number of VEGFR2/VE-PTP complexes at cell–cell junctions increased with VEGF+Ang1 ( Fig. 4f ). Furthermore, in cells silenced for tie2, VEGFR2/VE-PTP complex formation was reduced and insensitive to VEGF ( Fig. 4g ). These data strengthen the notions that Tie2 modulates VE-PTP’s interaction with VEGFR2 and that the three components communicate to balance quiescence preferentially at cell–cell junctions. VE-PTP in EC polarization and vessel lumen formation We observed a reduced number of pericytes associated with angiogenic sprouts in ve-ptp −/− EBs ( Supplementary Fig. S1a,b ); a hallmark of vessel immaturity. We therefore asked whether excess VEGFR2 activity in the absence of VE-PTP would interfere with vessel maturation. In WT sprouts at day 14 of differentiation, the apical/lumen markers podocalyxin and moesin [32] , [33] were detected at stalk EC junctions, which contained a clearly distinguishable lumen ( Fig. 5a , left). In ve-ptp −/− sprouts, podocalyxin and moesin were disorganized, surrounding certain ECs cells and missing from others ( Fig. 5a , right). Strikingly, ve-ptp −/− sprouts did not enclose a lumen but often presented a cup-shaped structure (see stalk cell image in Fig. 5a , right). About 25% of ve-ptp −/− ECs showed abnormally located podocalyxin ( Fig. 5b ) as determined in a double-blind assessment. 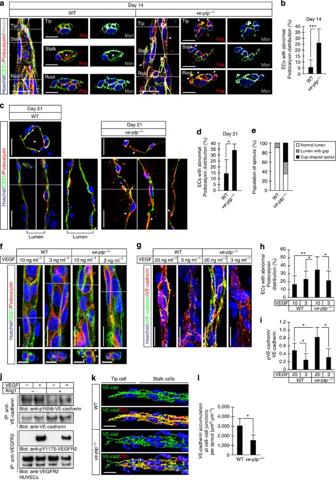Figure 5: VE-PTP is required for EC polarization and lumen formation. Panelsa,c,f,gandkshow immunostaining of WT andve-ptp−/−EBs at day 14 or 21, treated with 20 ng ml−1of VEGF or, when indicated, 3 ng ml−1. Hoechst 33342 (blue) staining shows nuclei. Dashed lines show position of parallel vertical-view images. (a) Podocalyxin (Pdx; red), moesin (Msn; white), CD31 (green). Scale bars, 20 μm. Vertical-view images represent sprout tip, stalk and root; scale bars, 10 μm. Asterisk, lumen; arrowhead, abnormal podocalyxin distribution. (b) Quantification of ECs with abnormal podocalyxin per total ECs ina. Mean±s.d.,n= 25 sprouts per genotype. ***P<0.001,t-test. (c) CD31 (green) and podocalyxin (red), show lumen in WT (asterisk) but cup-shapedve-ptp−/−sprouts. Scale bars, 20 μm. (d) Quantification of abnormal podocalyxin/total CD31+ECs in day 21 EBs. Mean±s.d.;n= 6 sprouts per genotype. *P<0.05,t-test. (e) Quantification of sprouts with continuous or discontinuous lumen and cup-shaped sprouts in the WT andve-ptp−/−EBs. Mean±s.d.;n=10 sprouts/WT EBs and 20/ve-ptp−/−EBs. (f) CD31 (green) and podocalyxin (red) in EBs treated with different concentrations of VEGF. Arrowheads, abnormal podocalyxin distribution. Scale bars, 20 μm. (g) pY658 VE-cadherin (green) and VE-cadherin (red) in EBs treated with different concentrations of VEGF. Scale bars, 20 μm. (h) Quantification of ECs with abnormally localized podocalyxin inf. Mean±s.d.;n= 14–15 sprouts for each condition, *P<0.05, **P<0.01,t-test. (i) Quantification of pVE-cadherin/VE-cadherin ing. Mean±s.d.;n= 5–8 sprouts for each condition, *P<0.05,t-test. (j) HUVECs treated individually with VEGF, Ang1 or VEGF+Ang1, immunoprecipitation (IP) of VE-cadherin and VEGFR2, and immunoblotting for pY658 VE-cadherin, VE-cadherin, pY1175 VEGFR2 and VEGFR2. (k) WT andve-ptp−/−EBs at day 14 represented by 3D Imaris images show VE-cadherin (VE-cad; green) and ZO1 (red). Arrows, fragmented VE-cadherin. Scale bars, 20 μm. (l) Quantification of VE-cadherin colocalized with ZO1 per 100 μm sprout length. Mean±s.d.n=4 sprouts for each condition. *P<0.05,t-test. Figure 5: VE-PTP is required for EC polarization and lumen formation. Panels a , c , f , g and k show immunostaining of WT and ve-ptp −/− EBs at day 14 or 21, treated with 20 ng ml −1 of VEGF or, when indicated, 3 ng ml −1 . Hoechst 33342 (blue) staining shows nuclei. Dashed lines show position of parallel vertical-view images. ( a ) Podocalyxin (Pdx; red), moesin (Msn; white), CD31 (green). Scale bars, 20 μm. Vertical-view images represent sprout tip, stalk and root; scale bars, 10 μm. Asterisk, lumen; arrowhead, abnormal podocalyxin distribution. ( b ) Quantification of ECs with abnormal podocalyxin per total ECs in a . Mean±s.d., n = 25 sprouts per genotype. *** P <0.001, t -test. ( c ) CD31 (green) and podocalyxin (red), show lumen in WT (asterisk) but cup-shaped ve-ptp −/− sprouts. Scale bars, 20 μm. ( d ) Quantification of abnormal podocalyxin/total CD31 + ECs in day 21 EBs. Mean±s.d. ; n = 6 sprouts per genotype. * P <0.05, t -test. ( e ) Quantification of sprouts with continuous or discontinuous lumen and cup-shaped sprouts in the WT and ve-ptp −/− EBs. Mean±s.d. ; n =10 sprouts/WT EBs and 20/ ve-ptp −/− EBs. ( f ) CD31 (green) and podocalyxin (red) in EBs treated with different concentrations of VEGF. Arrowheads, abnormal podocalyxin distribution. Scale bars, 20 μm. ( g ) pY658 VE-cadherin (green) and VE-cadherin (red) in EBs treated with different concentrations of VEGF. Scale bars, 20 μm. ( h ) Quantification of ECs with abnormally localized podocalyxin in f . Mean±s.d. ; n = 14–15 sprouts for each condition, * P <0.05, ** P <0.01, t -test. ( i ) Quantification of pVE-cadherin/VE-cadherin in g . Mean±s.d. ; n = 5–8 sprouts for each condition, * P <0.05, t -test. ( j ) HUVECs treated individually with VEGF, Ang1 or VEGF+Ang1, immunoprecipitation (IP) of VE-cadherin and VEGFR2, and immunoblotting for pY658 VE-cadherin, VE-cadherin, pY1175 VEGFR2 and VEGFR2. ( k ) WT and ve-ptp −/− EBs at day 14 represented by 3D Imaris images show VE-cadherin (VE-cad; green) and ZO1 (red). Arrows, fragmented VE-cadherin. Scale bars, 20 μm. ( l ) Quantification of VE-cadherin colocalized with ZO1 per 100 μm sprout length. Mean±s.d. n =4 sprouts for each condition. * P <0.05, t -test. Full size image At day 21 of differentiation, the WT sprouts displayed lumens encompassed by 2–3 ECs ( Fig. 5c ). ve-ptp −/− sprouts on the other hand showed cup-shaped EC formations with disorganized podocalyxin/moesin immunostaining ( Fig. 5d ). Inspection of sprouts for i) continuous lumen formation along the sprout length, ii) the presence of occasional gaps or iii) cup-shaped sprouts, showed that only 30% of the ve-ptp −/− sprouts contained a continuous lumen compared with 90% of WT sprouts ( Fig. 5e ). Importantly, the frequency of ECs with abnormal podocalyxin distribution decreased with decreased VEGF levels in the EB cultures (3 ng ml −1 ; Fig. 5f ). Furthermore, phosphorylation of Y658 in VE-cadherin was high in VEGF-treated ve-ptp −/− EBs (20 ng ml −1 ; Fig. 5g ), and lowering the dose to 3 ng ml −1 VEGF rescued pVE-cadherin levels to that of WT EBs ( Fig. 5g ). Figure 5h show quantification of podocalyxin distribution and pVE-cadherin levels in EBs treated with different concentrations of VEGF. In primary ECs, pY658 VE-cadherin levels increased with VEGF stimulation and decreased again when cells were treated with VEGF+Ang1 ( Fig. 5j ), implicating VE-PTP in regulation of pY658 VE-cadherin. Increased pY658 VE-cadherin was accompanied by reduced localization of VE-cadherin in ZO1-positive junctions in the ve-ptp −/− sprouts ( Fig. 5k ). Combined, these data indicate that VE-PTP deficiency resulted in increased phosphorylation of VE-cadherin accompanied by polarization and lumen defects, in a manner that could be rescued by limiting VEGFR2 activation. To further define the role of Ang1/Tie2 in EC polarization and lumen formation, we treated WT EBs with a Tie2-extracellular domain soluble protein (sTie2/Fc) to neutralize endogenous Ang1 produced by the cultures. We hypothesized that blocking Ang1 using sTie2/Fc would suppress the capacity of VE-PTP to dephosphorylate VEGFR2. Indeed, podocalyxin was broadly distributed and surrounded ECs in sTie2/Fc-treated EBs, whereas untreated EB sprouts displayed polarized, apical distribution of podocalyxin ( Fig. 6a ). Furthermore, the sTie2/Fc-treated vessel sprouts showed reduced capacity to lumenize. In agreement with a role for VEGFR2 in this process, WT EBs treated with sTie2/Fc showed increased levels of both VEGFR2 and pVEGFR2, and the pVEGFR2/VEGFR2 ratio was elevated in the stalk region ( Fig. 6c ). These data show that neutralization of endogenously expressed Ang1 ( Fig. 6e ) by the sTie2/Fc phenocopied the effect of ve-ptp targeting, resulting in elevated pVEGFR2 activity and unpolarized vessels with lumen defects. Therefore, even though VEGF and Ang1 did not regulate the extent of formation of the trimeric complex ( Fig. 2i ), Ang1 appeared critical in junctional translocation of the complex. 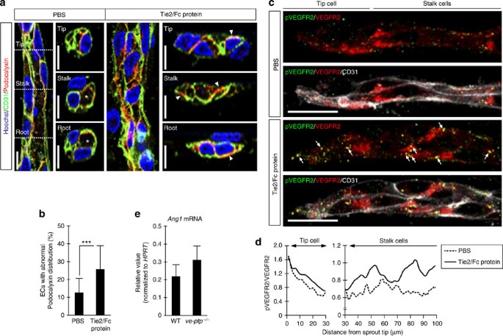Figure 6: Tie2 is required in VE-PTP-mediated VEGFR2 dephosphorylation. (a) WT EBs in 3D collagen with VEGF (20 ng ml−1) in the presence or absence of Tie2/Fc protein (4 μg ml−1) show CD31 (green), podocalyxin (red) and Hoechst 33342 (blue). Dashed lines show position of vertical-view images displayed in panels labelled tip, stalk and root. Scale bars, 10 μm. Asterisk, lumen; arrowhead, abnormal podocalyxin distribution. (b) Quantification of ECs with abnormal podocalyxin distribution. Mean±s.d.,n= 20 sprouts per condition. ***P<0.001,t-test. (c) pVEGFR2 (green), VEGFR2 (red) and CD31 (white) at day 14 in WT EBs treated or not with Tie2/Fc protein (4 μg ml−1). Arrows indicate pVEGFR2. Scale bars; 20 μm. (d) Ratio of pVEGFR2/VEGFR2 intensities from sprout tip to stalk. Data show the mean;n= 8 sprouts/condition. (e) Ang1 transcript expression/HPRT expression in WT andve-ptp−/−EBs in 2D collagen with VEGF (20 ng ml−1) at day 14. Mean±s.d. Statistics are based on two independent experiments withn=150 EBs per experiment. Figure 6: Tie2 is required in VE-PTP-mediated VEGFR2 dephosphorylation. ( a ) WT EBs in 3D collagen with VEGF (20 ng ml −1 ) in the presence or absence of Tie2/Fc protein (4 μg ml −1 ) show CD31 (green), podocalyxin (red) and Hoechst 33342 (blue). Dashed lines show position of vertical-view images displayed in panels labelled tip, stalk and root. Scale bars, 10 μm. Asterisk, lumen; arrowhead, abnormal podocalyxin distribution. ( b ) Quantification of ECs with abnormal podocalyxin distribution. Mean±s.d., n = 20 sprouts per condition. *** P <0.001, t -test. ( c ) pVEGFR2 (green), VEGFR2 (red) and CD31 (white) at day 14 in WT EBs treated or not with Tie2/Fc protein (4 μg ml −1 ). Arrows indicate pVEGFR2. Scale bars; 20 μm. ( d ) Ratio of pVEGFR2/VEGFR2 intensities from sprout tip to stalk. Data show the mean; n = 8 sprouts/condition. ( e ) Ang1 transcript expression/HPRT expression in WT and ve-ptp −/− EBs in 2D collagen with VEGF (20 ng ml −1 ) at day 14. Mean±s.d. Statistics are based on two independent experiments with n =150 EBs per experiment. Full size image To provide in vivo confirmation of a role for VE-PTP in vessel lumen formation, we used WT and ve-ptp −/− ESCs to establish teratomas in severe combined immunodeficient (SCID) mice. Teratomas become vascularized in part from the host and in part through differentiation of ECs from the ESCs [34] . As shown in Fig. 7a , vessels in ve-ptp −/− teratomas displayed disorganized ECs with broadly distributed podocalyxin expression ( Fig. 7a ). Immunostaining for pVEGFR2 moreover demonstrated significant induction of VEGFR2 phosphorylation in CD31-positive ECs in ve-ptp −/− teratomas ( Fig. 7c ). Co-immunostaining for pVEGFR2 and VE-PTP showed that ECs in perfused, lumenized vessels in WT teratomas expressed VE-PTP, but displayed very low levels of pVEGFR2. In contrast, disorganized and poorly perfused vessels in ve-ptp −/− teratomas, which we confirmed lacked expression of VE-PTP, displayed prominent pVEGFR2 immunostaining ( Fig. 7e ). Omitting the primary antibody demonstrated the specificity of the immunostainings ( Fig. 7e ). There was furthermore a correlation between the extent of perfusion, the expression of VE-PTP and the ordered arrangement of VE-cadherin in the WT teratomas. In non-perfused vascular structures in the ve-ptp −/− teratomas, the VE-cadherin pattern appeared fragmented ( Fig. 7f ). We also analysed VE-PTP expression in B16 F10 melanoma and identified a correlation between perfusion (functionality), VE-PTP expression and continuous VE-cadherin immunostaining on the one hand, and lack of perfusion, lack of VE-PTP expression and fragmented VE-cadherin on the other hand ( Fig. 7g ). Our data support a model in which Tie2-mediated suppression of VEGFR2 activity at EC junctions through VE-PTP is essential for formation of functional vessels. In pathological conditions characterized by excess VEGF production and faulty expression VE-PTP, ECs fail to polarize, which leads to a poorly functional vasculature with partially or completely collapsed lumen ( Fig. 7h ). 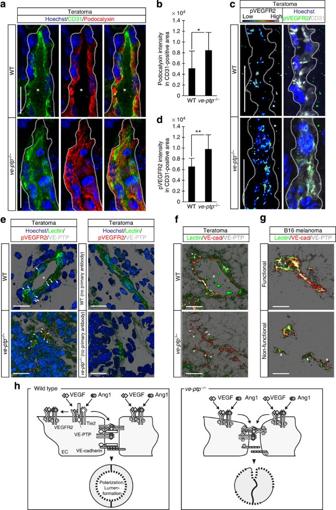Figure 7: VE-PTP regulates VEGFR2 activity and polarizationin vivo. (a) WT andve-ptp−/−teratoma sections show CD31 (green), podocalyxin (red) and Hoechst 33342 (blue). Asterisk, lumen. Scale bars, 20 μm. (b) Podocalyxin intensity/CD31-positive area (mm3) ina. Mean±s.d.;n= 15 CD31-positive vessels of 50 μm length/3 teratomas/genotype. *P<0.05,t-test. (c) WT andve-ptp−/−teratoma sections. Left: 16-colour intensity scale representation of pVEGFR2 immunostaining. Right: Hoechst 33342 (blue), pY1175 VEGFR2 (green), and CD31 (grey). Scale bars, 20 μm. (d) pY1175 VEGFR2 intensity/CD31-positive area (mm2) inc. Mean±s.d.;n= 12 (WT) and 15 (ve-ptp−/−) blood vessels of 30 μm length from 3 teratomas per genotype. **P<0.01,t-test. (e) Lectin-perfused WT andve-ptp−/−teratomas. Hoechst 33342 (blue), lectin-FITC (green), pY1175 VEGFR2 (red) and VE-PTP (white). Right: control immunostaining without primary antibodies. Asterisk, lumen. Arrows show VE-PTP expression in WT teratomas. Arrowheads show pVEGFR2 inve-ptp−/−teratomas. Scale bars, 20 μm. (f) Lectin-perfused WT andve-ptp−/−teratomas show lectin-FITC (green), VE-cadherin (red) and VE-PTP (white). Asterisk, lumen. Arrowheads in the lowerve-ptp−/−panel indicate fragmented VE-cadherin immunostaining. Scale bars, 20 μm. (g) Lectin-perfused B16 F10 mouse melanomas show lectin-FITC (green), VE-cadherin (VE-cad; red) and VE-PTP (white). Asterisk, lumen. Arrowheads in the lower panel indicate fragmented VE-cadherin immunostaining. Scale bars, 20 μm. (h) Model illustrating the contribution of VE-PTP in silencing VEGFR2 and Tie2 at junctions to support proper EC polarity and vessel morphogenesis. VE-PTP exists in complex with VEGFR2 and Tie2 in the WT condition (left). VEGF induces activation of VEGFR2 and in parallel, dissociation from VE-PTP. VEGF and Ang1 induce translocation of the trimeric complex to junctions where the activated receptors are silenced by VE-PTP. This is compatible with formation of polarized and lumenized vessels. In the VE-PTP-deficient condition (ve-ptp−/−; right), VEGF and Ang1 induce activation and translocation of receptors to junctions, where excess activity leads to VE-cadherin phosphorylation and formation of unpolarized and lumen-less pathological vasculature. Figure 7: VE-PTP regulates VEGFR2 activity and polarization in vivo. ( a ) WT and ve-ptp −/− teratoma sections show CD31 (green), podocalyxin (red) and Hoechst 33342 (blue). Asterisk, lumen. Scale bars, 20 μm. ( b ) Podocalyxin intensity/CD31-positive area (mm 3 ) in a . Mean±s.d. ; n = 15 CD31-positive vessels of 50 μm length/3 teratomas/genotype. * P <0.05, t -test. ( c ) WT and ve-ptp −/− teratoma sections. Left: 16-colour intensity scale representation of pVEGFR2 immunostaining. Right: Hoechst 33342 (blue), pY1175 VEGFR2 (green), and CD31 (grey). Scale bars, 20 μm. ( d ) pY1175 VEGFR2 intensity/CD31-positive area (mm 2 ) in c . Mean±s.d. ; n = 12 (WT) and 15 ( ve-ptp −/− ) blood vessels of 30 μm length from 3 teratomas per genotype. ** P <0.01, t -test. ( e ) Lectin-perfused WT and ve-ptp −/− teratomas. Hoechst 33342 (blue), lectin-FITC (green), pY1175 VEGFR2 (red) and VE-PTP (white). Right: control immunostaining without primary antibodies. Asterisk, lumen. Arrows show VE-PTP expression in WT teratomas. Arrowheads show pVEGFR2 in ve-ptp −/− teratomas. Scale bars, 20 μm. ( f ) Lectin-perfused WT and ve-ptp −/− teratomas show lectin-FITC (green), VE-cadherin (red) and VE-PTP (white). Asterisk, lumen. Arrowheads in the lower ve-ptp −/− panel indicate fragmented VE-cadherin immunostaining. Scale bars, 20 μm. ( g ) Lectin-perfused B16 F10 mouse melanomas show lectin-FITC (green), VE-cadherin (VE-cad; red) and VE-PTP (white). Asterisk, lumen. Arrowheads in the lower panel indicate fragmented VE-cadherin immunostaining. Scale bars, 20 μm. ( h ) Model illustrating the contribution of VE-PTP in silencing VEGFR2 and Tie2 at junctions to support proper EC polarity and vessel morphogenesis. VE-PTP exists in complex with VEGFR2 and Tie2 in the WT condition (left). VEGF induces activation of VEGFR2 and in parallel, dissociation from VE-PTP. VEGF and Ang1 induce translocation of the trimeric complex to junctions where the activated receptors are silenced by VE-PTP. This is compatible with formation of polarized and lumenized vessels. In the VE-PTP-deficient condition ( ve-ptp −/− ; right), VEGF and Ang1 induce activation and translocation of receptors to junctions, where excess activity leads to VE-cadherin phosphorylation and formation of unpolarized and lumen-less pathological vasculature. Full size image Zebrafish ptp-rb in EC polarization and lumen formation We further explored VE-PTP's role in EC polarization and lumen formation in the zebrafish embryo. Formation of trunk intersomitic vessels (ISVs) in the zebrafish occurs through sprouting angiogenesis in a VEGF-dependent manner [35] , [36] , [37] , [38] . We first cloned the zebrafish VE-PTP orthologue, by searching for zebrafish sequences homologous to the mouse (m) VE-PTP catalytic domain. We identified a gene here denoted as ptp-rb , that we showed by in situ hybridization was expressed in ISVs during development ( Supplementary Fig. S6 ). The corresponding protein is composed of fibronectin type III repeats repeats in the extracellular domain and a typical PTP catalytic intracellular domain. The catalytic domain of ptp-rb showed a striking degree of homology to murine VE-PTP with all catalytic PTP motifs presented. Two morpholinos (MOs) were used to specifically knock-down ptp-rb expression in the Tg(fli1a:EGFP) y1 transgenic background, where vascular endothelia express GFP [39] . The specificity of the ptp-rb MOs was verified by cloning of the resulting PCR fragment from MO-injected embryos ( Supplementary Fig. S6d,e ). In the 48-h post-fertilization embryos, control MO-treated ISVs displayed a characteristic chevron morphology and were lumenized. In contrast, in ptp-rb morphants, many ISVs had abnormal morphology and often lacked a continuous lumen ( Fig. 8a–c ). The number of embryos with ISV defects as well as the number of ISV defects per embryo significantly decreased by co-injecting the ptp-rb MO with human ptp-rb ( ve-ptp ) RNA, demonstrating that the vascular defects were due to loss of zebrafish ptp-rb function ( Supplementary Fig. S7a–c ). ptp-rb MO-treated ISVs failed to form a patent lumen ( Fig. 8b ); there was a twofold increase in lumen-less vessels/embryo when ptp-rb expression was suppressed ( Fig. 8c ). In accordance, double transgenic Tg(kdrl:EGFP) s843 ; Tg(gata1:dsRed) sd2 embryos showed flow in the control MO-treated embryos from the dorsal aorta (DA) through the ISVs to the dorsal longitudinal anastomosing vessel (DLAV), whereas embryos treated with ptp-rb MOs lacked dsRed-positive cells in the DLAV ( Supplementary Fig. S7d ); see also Supplementary Movies 1 and 2. This finding supports the notion that the majority of the ptp-rb -deficient ISVs lacked lumen, thereby preventing circulation through the ISV to the DLAV. In contrast, the ptp-rb -deficient DA contained blood cells, indicating that lumen formation in ISVs, which is established through sprouting angiogenesis, is distinct from lumenization of the DA during vasculogenesis. 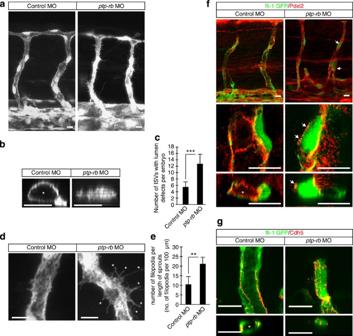Figure 8: Zebrafishptp-rbregulates ISV lumen formation. (a) At 48 hours post fertilization,ptp-rbMO ISVs migrate and anastomose to make a DLAV, but lack patent lumens and are covered with filopodia compared with control MO-treated embryos. Scale bars, 10 μm. (b) Transverse optical sections show lumen in control MO-treated ISV (asterisk), whereasptp-rbMO ISV lacks a lumen. Scale bars, 10 μm. (c) ISV lumen defects per embryo. Mean±s.d.,n=12 (control MO) and 10 (ptp-rbMO) embryos. ***P<0.001,t-test. (d) Close-up view of theptp-rbMO hyperfilopodial phenotype. Scale bars, 10 μm. (e) Quantification of number of filopodia per 10 μm. Mean±s.d.;n= 4 (control MO) and 7 (ptp-rbMO) ISVs. **P<0.01,t-test. (f) Podocalyxin (Pdxl; red) in control andptp-rbMO-treated embryos. Upper, middle and lower panels show overviews, high-magnification and transvere images of ISVs, respectively. Asterisk, lumen; arrows indicate Podocalyxin mislocalization. Scale bars, 10 μm. (g) VE-cadherin (Cdh5; red) in ISVs (upper) in control andptp-rbMO-treated embryos. Lower panels show transverse images of ISVs. Blood vessels are defined byfli-1promoter-driven GFP (green) infandg. Scale bars, 10 μm. Figure 8: Zebrafish ptp-rb regulates ISV lumen formation. ( a ) At 48 hours post fertilization, ptp-rb MO ISVs migrate and anastomose to make a DLAV, but lack patent lumens and are covered with filopodia compared with control MO-treated embryos. Scale bars, 10 μm. ( b ) Transverse optical sections show lumen in control MO-treated ISV (asterisk), whereas ptp-rb MO ISV lacks a lumen. Scale bars, 10 μm. ( c ) ISV lumen defects per embryo. Mean±s.d., n =12 (control MO) and 10 ( ptp-rb MO) embryos. *** P <0.001, t -test. ( d ) Close-up view of the ptp-rb MO hyperfilopodial phenotype. Scale bars, 10 μm. ( e ) Quantification of number of filopodia per 10 μm. Mean±s.d. ; n = 4 (control MO) and 7 ( ptp-rb MO) ISVs. ** P <0.01, t -test. ( f ) Podocalyxin (Pdxl; red) in control and ptp-rb MO-treated embryos. Upper, middle and lower panels show overviews, high-magnification and transvere images of ISVs, respectively. Asterisk, lumen; arrows indicate Podocalyxin mislocalization. Scale bars, 10 μm. ( g ) VE-cadherin (Cdh5; red) in ISVs (upper) in control and ptp-rb MO-treated embryos. Lower panels show transverse images of ISVs. Blood vessels are defined by fli-1 promoter-driven GFP (green) in f and g . Scale bars, 10 μm. Full size image Cell counting in the Tg(fli1a:nEGFP) y7 transgenic background revealed no difference in the number of ISV ECs between ptp-rb MO-treated embryos and controls (data not shown). However, there was a significant increase in the number and density of long filopodia extending from the ISV ECs in the ptp-rb MO Tg(fli1a:nEGFP) y7 zebrafish ( Fig. 8d ). Immunostaining for podocalyxin in the control MO-treated fish embryos decorated the apical aspect of ECs, while ptp-rb MO-treated embryos showed a broad distribution and clear dysregulated polarity and lack of lumen ( Fig. 8f ). Immunostaining for zebrafish VE-cadherin (Cdh5) demonstrated a fragmented distribution and identified lumen-less vessels in the ptp-rb MO-treated embryos ( Fig. 8g ). Immunostaining for the tight junction protein ZO1 ( Supplementary Fig. S7e ) and the basement membrane component laminin, a marker for basal polarity ( Suppelmentary Fig. S7f ), further identified unpolarized, closed vessels in the absence of ptp-rb . Altogether, these data show that ptp-rb is essential for EC polarization and lumen formation in the zebrafish ISVs, demonstrating a conserved function of VE-PTP in zebrafish and mice. Here, we show that VE-PTP is crucial for EC polarization and lumen formation in angiogenic sprouts formed in EBs, in tumours and in ISVs in the developing zebrafish. The underlying mechanism involves VE-PTP-mediated dephosphorylation and thereby inactivation of VEGFR2 in EC junctions in an Ang1/Tie2-dependent manner. Tie2 serves as a direct substrate for VE-PTP, as a VE-PTP-trapping mutant binds Tie2 and protects it from dephosphorylation [26] . VE-PTP also dephosphorylates VE-cadherin and its robust interaction with VE-cadherin is mediated by the extracellular domains of both proteins, rather than by the phosphorylated intracellular domain [11] . Using in situ PLA, we identified VEGFR2 and VE-PTP complexes that formed in the presence of Tie2, indicating that the complexes contain all three components; VE-PTP, VEGFR2 and Tie2. The existence of a trimeric complex was demonstrated using consecutive immunoprecipitation and blotting ( Fig. 2i ). We also identified complexes composed of Tie2 and VEGFR2, which in response to VEGF treatment contained active VEGFR2 ( Fig. 2i ). The complexes are therefore likely to contain dimeric constellations of the receptor tyrosine kinases. Full-length VE-PTP failed to engage in complex formation and dephosphorylate either Tie2 or VEGFR2 using purified protein preparations (data not shown). The structural constraint but also specificity was overcome when using a truncated VE-PTP catalytic domain that dephosphorylated VEGFR2 in a Tie2-independent manner in vitro ( Supplementary Fig. S2b ). These data indicate that formation of the trimeric complex affects folding of at least VE-PTP to allow its in vivo activity towards Tie2 and indirectly, towards VEGFR2. The phosphatase activity of VE-PTP towards VEGFR2 was independent of Tie2 kinase activity. We suggest that the ligands, VEGF and Ang1, instead are essential in transport of the complex to endothelial junctions (see schematic outline; Fig. 7h ). In response to VEGF, the number of VE-PTP/receptor complexes detected by PLA decreased overall in the cell, but increased at junctions ( Fig. 4d–f ). In agreement, ve-ptp silencing preferentially increased the junctional localization of active VEGFR2 ( Fig. 4a ). These data suggest that VE-PTP has to dissociate from the receptor to allow tyrosine kinase activation but that VE-PTP acts as a safe guard at junctions to maintain quiescence. We do not exclude that the overall decrease in VE-PTP/VEGFR2 complexes in response to VEGF is due to, for example, internalization and degradation. However, as Tie2 silencing desensitized VE-PTP/VEGFR2 complexes from the effect of VEGF ( Fig. 4g ), we favour a model where VEGF-induced activation of VEGFR2 requires dissociation from VE-PTP. VE-PTP has thus far been shown to dephosphorylate Tie2, VE-cadherin and plakoglobin, which all are localized to EC–cell junctions, transiently or constitutively [14] , [40] . Immunostaining showed preferential localization of VE-PTP at cell–cell junctions ( Fig. 1h ). Accordingly, depletion of VE-PTP leads to weakening of EC junctions [12] . The subcellular localization of VEGFR2 in different angiogenic stages has not been dissected. However, the fact that VEGFR2 occurs in complex with VE-cadherin [17] strongly indicates localization of at least part of the VEGFR2 pool at junctions. Furthermore, we show that in confluent, but not sparse, cultures of primary ECs, combined VEGF/Ang1 treatment suppresses active VEGFR2 at junctions ( Fig. 3 ). Tie2/VE-PTP complexes occur also outside cell–cell junctions [10] . Whether VEGFR2/VE-PTP complexes are established in junctions or, alternatively, outside junctions followed by ligand-mediated translocation to junctions, remains to be firmly established. Thus, we do not exclude a dynamic situation where complexes form and dissolve, or become internalized, outside junctions. Lumen formation in the mouse DA, and in mouse arteries, is preceded by establishment of endothelial polarity [15] , [32] , [41] , [42] . In immature vessel cords lacking a patent lumen, VE-cadherin is distributed throughout the entire cell–cell contact area of adjacent plasma membranes [32] . Subsequently, VE-cadherin becomes relocalized laterally and the lumen opens up, guided by strictly regulated cell shape changes. VE-cadherin-deficient mice show impaired lumen formation followed by EC apoptosis [17] . We show that excess VE-cadherin phosphorylation at Y658 also interferes with cell polarization and lumen formation, stressing the important role of balanced VE-cadherin biology and tyrosine kinase activity at the junction. The fact that lowering the VEGF dose in the EB cultures rescued cell polarity and lumen formation in the ve-ptp −/− sprouts suggests that dysregulated VEGFR2 activity in endothelial junctions is a primary defect in the ve-ptp −/− condition. Bäumer et al . [9] reported normal morphology of EC junctions in enlarged vessels of the yolk sac of ve-ptp -targeted mice. By analysis of phoshorylation of VE-cadherin at Y658, we show increased phosphorylation levels in the absence of VE-PTP, indicating immature and therefore unstable junctions in sprouts of EBs. Morphologically, VE-PTP deficiency was accompanied by a fragmented appearance of VE-cadherin immunostaining. Disturbances in other steps of the polarization process in ve-ptp -deficient ECs, such as the communication with the extracellular matrix [41] , or defects in the partitioning-defective (PAR) polarity complex [43] , [44] , [45] , [46] , [47] may have contributed to the polarity and lumen formation abnormalities. Silencing of the ve-ptp orthologue in zebrafish, denoted ptp-rb , allowed lumenization of the DA, which forms through vasculogenesis, but not of the ISVs, which form through sprouting angiogenesis. That VE-PTP is dispensable for essential aspects of vasculogenesis also in the mouse is in accordance with that its expression is induced after onset of vasculogenesis and that it is required for remodelling rather than establishment of the vascular plexus [8] , [9] . Ang1/Tie2 has been implicated in stabilization and maturation of growing blood vessels [48] , [49] , and Ang1 efficiently blocks VEGF-induced EC permeability in vitro [50] and in vivo [49] . A signalling chain involving RhoA, mDIA and sequestration of Src (ref. 51 ) has been implicated in the vessel-stabilizing effect of Ang1/Tie2. Here, we show how Tie2 mediates suppressed VEGFR2 activity at EC junctions through VE-PTP ( Fig. 7h ), providing an important mechanism for the molecular communication between Ang1/Tie2 and VEGF/VEGFR2 in formation and maintenance of a functional vasculature. Cells Human umbilical vein ECs (HUVECs; American Type Tissue Collection) were seeded in sparse (5,000 cells per cm 2 ) or confluent (50,000 cells per cm 2 ) conditions. HUVECs starved in MV2 medium with 1% FCS for 2 h-overnight were stimulated with 20 ng ml −1 of mouse VEGF-A164 (PeproTech), 200 ng ml −1 of COMP-Angiopoietin-1 (COMP-Ang1) [52] , or both, for time periods indicated. When indicated, human VEGFC (PeproTech) was used at 200 ng ml −1 . PAE cells expressing human VEGFR2 (PAE/VEGFR2 (ref. 53 )) and PAE/VEGFR3 ( 54 ), were maintained in Ham’s F12 (Invitrogen), 10% FCS. Human embryonic kidney 293T cells were maintained in DMEM (Invitrogen), 10% FCS. For transient transfections, cells were seeded on 6-well plates and transfected using Lipofectamin 2000 (Invitrogen). Gene-targeted ve-ptp −/− ESCs were established using the VelociGene strategy [55] . ESCs were differentiated to create EBs, in two or three-dimensional (2D or 3D) cultures [21] and treated with 3, 10, 20 ng ml −1 of mVEGF-A164, 200 ng ml −1 of COMP-Ang1 or both. When indicated, mouse Tie2/Fc chimeric protein (final concentration; 4 μg ml −1 , R&D Systems) was added. Antibodies Antibodies for immunofluorescence: anti-mouse CD31 (BD Biosciences), anti-mouse NG2 (Millipore), anti-mouse Podocalyxin (R&D Systems), anti-mouse Moesin (Abcam), anti-mouse VE-cadherin (BD Biosciences), anti-VE-PTP (hPTPb1-8) (ref. 10 ), anti-mouse VEGFR2 (R&D Systems), anti-human VEGFR2 (R&D Systems), anti-human pY1175 VEGFR2 (Cell Signaling), anti-human Tie2 (R&D Systems), anti-VE-cadherin (BD Biosciences) and anti-pY658 VE-cadherin [31] . Conjugated secondary antibodies: Alexa-488, Alexa-555, Alexa-647 (Invitrogen) and Cy5 (Jackson ImmunoResearch Laboratories). Hoechst 33342 was used to visualize nuclei. Antibodies for immunoprecipitation/immunoblotting: Anti-V5 (Invitrogen), anti-human pY992 Tie2 (Cell Signaling), anti-human Tie2, anti-human VEGFR2, anti-human pY1175 VEGFR2, anti-human VEGFR3, anti-human Tie1, anti-human VE-PTP and anti-human α-actin (Santa Cruz Biotechnology). Antibodies for PLA reactions: anti-human VEGFR2 (R&D Systems and Cell Signaling), anti-human Tie2, anti-VE-PTP and anti-pY1175 VEGFR2. Samples were analysed using a Nikon Eclipse E1000 microscope (Nikon) with a Hamamatsu Digital Camera C10600 (Hamamatsu), a LSM 510 META or a LSM 700 confocal microscope (Carl Zeiss). Sequential immunoprecipitation/immunoblotting Analyses repeated three times and representative results are shown. Quantification of immunoblotting was done using ImageJ (NIH). For sequential immunoprecipitation, the first precipitate with anti-FLAG antibody was eluted from protein G-Sepharose beads with 0.1 M glycine-HCl, pH 3.4, neutralized to pH 7.4, followed by the second immunoprecipitation with anti-V5 antibody; the supernatant was immunoprecipitated with anti-VEGFR2 antibodies. Samples were processed further by immunoblotting as indicated. Plasmids Human VE-PTP complementary DNA was subcloned into pcDNA/V5/GW/D-TOPO Vector. A substrate-trapping mutant of VE-PTP (replacement of aspartic acid 1180 in the catalytic domain for alanine) was generated by nested PCR. The following primers were used to generate two sets of PCR amplicons. For the first set; forward primer 1, 5′-TTTGGTACC TGGTGTCCA TCAAAGTGCA-3′ and reverse primer 1, 5′-CTGGGACTCCATGGGCTGGCCACACCGT-3′. For the second set; forward primer 2, 5′-ACGGTGTGGCCAGACCATGGAGTCCCAG-3′ and reverse primer 2, 5′-TTTGCTAGCCTAACCGGTACGCGTAGA-3′. Using the two amplicons of the first PCR as templates, the forward primer from the first set and the reverse primer from the second set were used for the second PCR. Expression vectors for Tie2-FLAG (that is, Tie2 fused C-terminally with the peptide DYKDDDDK) and Tie2 intracellular domain-truncated mutant were described previously [56] . A kinase-dead mutant of human Tie2 (replacement of lysine 855 for alanine) [22] was generated by GeneArt Site-Directed Mutagenesis System (Invitrogen). The Tie2-FLAG expression vector was used as a template. The following primers were used; 5′-CGGATGGATGCTGCCATCGCCAGAATGAAAGAATATGCCTCC-3′ and 5′-GGAGGCATATTCTTTCATTCTGGCGATGGCAGCATCCATCCG-3′. siRNA transfection HUVECs were transfected using Lipofectamine RNAiMax (Invitrogen) with Stealth RNA duplex oligoribonucleotides against human VE-PTP (HSS108847; Invitrogen), human Tie2 (HSS110624; Invitrogen), human Tie1 (HSS110624 and HSS110625; Invitrogen) or control siRNA (12935-300; Invitrogen). RNA extraction, cDNA synthesis and quantitative real-time PCR (qRT–PCR) analysis EBs (50 EBs per dish) were cultured in 2D condition with or without 20 ng ml −1 of VEGF. At day 14, CD31-positive cells were isolated using magnetic cell sorting (MACS; (ref. 57 )). Magnetic beads were removed from the MACS-purified cell suspension using QIAshellder columns (Qiagen). Total RNAs were extracted using RNeasy Mini Kit (Qiagen). cDNAs were synthesized using 250 ng of total RNA, random primers (Invitrogen) and SuperScript III (Invitrogen). qRT–PCR was performed on cDNA using TaqMan Universal PCR Master Mix (Applied Biosystems) by StepOnePlus real-time PCR sytem (Applied Biosystems). EBs cultured in 3D condition with 20 ng ml −1 of VEGF were lysed using TRIzol (Invitorgen), following by extraction of total RNAs and synthesis of cDNAs. qRT–PCR was performed on cDNA using SYBR Green PCR Master Mix (Applied Biosystems) by StepOnePlus real-time PCR sytem. The following primers were used; mHPRT; forward primer, 5′-CAAACTTTGCTTTCCCTGGT-3′, reverse primer, 5′-TTCGAGAGGTCCTTTTCACC-3′ and mAng1; forward primer, 5′-GCTGACAGATGTTGAGACCCAGGTA-3′, reverse primer, 5′-TGACGAGAAACCAAGCCTTGAAGGT-3′. The following pre-designed primers (Applied Biosystems) were used: mGAPDH; part number 4352932E. Fluorescence-activated cell sorting (FACS) analysis EBs cultured for 9 days were collagenase-dissociated followed by isolation of CD31-positive ECs using MACS [57] . Cells were incubated with anti-VE-cadherin antibodies (R&D Systems) and donkey anti-goat Cy5 (Invitrogen), or stained with rat anti-mouse CD31-phycoerythrin antibody (BD Biosciences). DAPI-negative, viable cells were analysed on a FACSVantageSE machine using FACSDiVa software (BD Biosciences). Image analysis phospho-VEGFR2 and total VEGFR2 Concentration gradients were measured along the sprout, starting from a manually marked tip, using software built around a Semper6p core (Synoptics Ltd, Cambridge, UK). For each individual layer in a Z series, both fluorophores were used to define sprout limits and saved in a binary image. The midline along the sprout was created using a 2D erode to skeleton operation on a maximum projected image (in z axis). The skeleton was automatically connected to the manually selected tip and all other branches of the midline were deleted, leaving a line running along the midline. A series of points at equal steps along the midline were generated. The sprout was then salami sliced by making each point on the midline the centre of a zone of influence (the area closest to each point). The average fluorescence of each fluorophore within each zone was taken from a cumulative Z projection, which holds the sum of the fluorescence. A second cumulative Z projection of the binary images of the sprout gave the volume of each zone of influence. The fluorescence was divided by area to give the mean fluorescence per unit volume from the tip along the sprout. Deconvolution of images stacks used optimized MLE (Huygens Pro, version 4.2.1p3, SVI, Netherlands) with a theoretical PSF and optimized signal-to-noise ratio. Proximity ligation assay HUVECs (50,000 cells per cm 2 ) were starved for 2 h in MV2 medium with 1% FCS, followed by stimulation with VEGF, Ang1 or VEGF+Ang1. Cells were fixed for 10 min at room temperature with 4% PFA, and permeabilized for 5 min with 0.2% Triton X-100/PBS. PLA was performed using Duolink in situ PLA (Olink Bioscience). In the primary antibody reaction, cells were incubated with the mixtures of primary antibodies: anti-Tie2/VE-PTP, anti-VEGFR2/VE-PTP or pVEGFR2/total VEGFR2, and anti-ZO1. In the amplification reaction, cells were incubated with the reaction mixture, and anti-mouse IgG-conjugated Alexa-488 (Invitrogen) for anti-ZO1. Samples were analysed using a LSM 510 META or a LSM 700 META confocal microscope (Carl Zeiss). Quantification of PLA spots was done using ImageJ (NIH). The total number of PLA spots and number of PLA spots close to cell–cell junctions (within 2.5 μm) were counted in ~50 cells per condition. Zebrafish husbandry Zebrafish were housed at the Karolinska Institute (Stockholm, Sweden) facility using standard protocols [55] . The following transgenic lines were used in this study: Tg(fli1a:EGFP) y1 ;Tg(gata1:dsRed) sd2 , Tg(kdrl:EGFP) s843 , Tg(kdrl:msna-EGFP) is1 (refs 39 , 58 , 59 , 60 ). MO knockdown Two zebrafish ptp-rb MOs, MO1; 5′-GAGGTTTTGCAGAGGCATGTCTTCC-3′ and MO2; 5′-TGCGGGCACTGAGAAGGAGAACATC-3′, (Gene Tools) were injected at 125 mM. MO-injected zebrafish embryos were maintained at 28 °C in standard E3 water supplemented with 0.003% phenyl-2-thiourea. Knockdown of ptp-rb expression with MO2 was confirmed by RT–PCR, using primers 5′-TGCGGAAGGAGACTTTGACT-3′ and 5′-TAGGGTTTCCCTGGTGTGAG-3′. Phenotypic consequences of MO knockdown were assessed between 24 and 72 hours post fertilization. Confocal images were taken on a Zeiss LSM700 microscope. Zebrafish immunostainings Whole-mount antibody staining of zebrafish embryos with anti-ZO1 (Sigma), anti-Pdxl and anti-Cdh5 antibodies [36] , [37] was performed using acetone permeabilization. For staining with the zebrafish anti-VE-Cadherin/Cdh5 antibody, embryos were fixed in 2% PFA/PBS/0.1% Tween (PBST), permeabilized in PBST/0.5% Triton X-100, and incubated in primary antibody-diluted 1:500 in PBST/5% normal goat serum/1% BSA/0.1% Triton X-100. Embryos were washed in PBST and stained with goat anti-rabbit or goat anti-mouse Alexa-568 secondary antibodies (Invitrogen). Images were collected on a Zeiss LSM 700 confocal microscope. Image analysis was done using ImageJ (NIH) and Imaris (Bitplane). In vivo tumour model WT or ve-ptp −/− ES cells (3 × 10 6 cells per 100 μl) were injected subcutaneously in the flank of SCID mice. Lectin-FITC (Fluorescein-conjugated ( FITC ) Lycopersicon esculentum (tomato) lectin (Vector Laboratories, Burlingame, CA, FL - 1171 ) was injected into the tail vein at day 24 after inoculation followed by harvesting of teratomas. Sections were analysed after immunofluorescent staining in a LSM 700 confocal microscope (Carl Zeiss), and quantified using Imaris (Bitplane). Mouse B16 melanoma cells (0.5 × 10 6 cells per 100μl) were injected subcutaneously in C57BL/6 mice and at day 12 after inoculation, animals were perfused with lectin-FITC injected in the tail vein. How to cite this article: Hayashi M. et al . VE-PTP regulates VEGFR2 activity in stalk cells to establish endothelial cell polarity and lumen formation. Nat. Commun. 4:1672 doi: 10.1038/ncomms2683 (2013).